Chemodiversity of dissolved organic matter in lakes driven by climate and hydrology Despite the small continental coverage of lakes, they are hotspots of carbon cycling, largely due to the processing of terrestrially derived dissolved organic matter (DOM). As DOM is an amalgam of heterogeneous compounds comprising gradients of microbial and physicochemical reactivity, the factors influencing DOM processing at the molecular level and the resulting patterns in DOM composition are not well understood. Here we show, using ultrahigh-resolution mass spectrometry to unambiguously identify 4,032 molecular formulae in 120 lakes across Sweden, that the molecular composition of DOM is shaped by precipitation, water residence time and temperature. Terrestrially derived DOM is selectively lost as residence time increases, with warmer temperatures enhancing the production of nitrogen-containing compounds. Using biodiversity concepts, we show that the molecular diversity of DOM, or chemodiversity, increases with DOM and nutrient concentrations. The observed molecular-level patterns indicate that terrestrially derived DOM will become more prevalent in lakes as climate gets wetter. Dissolved organic matter (DOM) is the major form of organic carbon in inland waters [1] , [2] and the oceans. In lakes, DOM is largely derived from terrestrial sources [3] and is central to food web dynamics [4] , [5] , [6] and global carbon cycling [7] , [8] . While oceans are the final receptacles of terrestrial DOM, transformations during transport through freshwater systems are important regulators of the ultimate quantity and quality of DOM delivered to marine systems [7] , [8] , [9] , [10] . Thus, controls on how inland waters process DOM are inherently linked to global biogeochemical cycling [7] , [8] , [9] . While many studies have sought to determine the drivers of DOM quality, developing a molecular-level understanding of DOM quality and dynamics has remained challenging due to its extreme heterogeneity. The burgeoning use of mass spectrometry in DOM studies has tremendously advanced our molecular-level understanding of DOM dynamics [11] , [12] , [13] , [14] , [15] . Recent developments in data processing now enable us to analyze the detailed molecular composition of DOM as a function of environmental gradients over a large number of samples. Ultrahigh-resolution electrospray ionization Fourier transform ion cyclotron resonance mass spectrometry (FT-ICR-MS) currently stands apart as the only method through which one can obtain detailed information on individual compounds in mixtures as complex as natural DOM. Thousands of molecular formulae are obtained for individual DOM compounds [16] from which basic structural features can be deduced, yielding a detailed illustration of the chemical diversity of the DOM. As the chemical composition of DOM constrains its microbial degradation [17] , chemodiversity may be useful in setting a baseline for the degradation potential of a system. Compounds range from photoreactive molecules like combustion-derived polycyclic aromatics, vascular plant-derived polyphenols, and highly unsaturated and phenolic compounds, to photoresistant aliphatic compounds and peptides [13] . Photoreactive compounds are often thought to be biologically recalcitrant, with aliphatic compounds and peptides being more bioavailable; however, allochthonous carbon has also been shown to be an important substrate for bacterial growth [18] , and photochemical transformations can enhance the bacterial mineralization of previously recalcitrant DOM [19] . Identifying the dynamics across these compound groups is central to understanding and predicting the reactivity and fate of DOM. We hypothesize that, in lakes, DOM molecular composition and diversity are related to broad-scale landscape and climatic variables. If confirmed, this information could be used to predict future changes in carbon processing across landscapes owing to changes in climate and land use. To this end, we first look at the distribution of dissolved organic molecules across 120 Swedish lakes, finding an abundant core of reoccurring molecules present in most lakes, with a long tail of rare compounds. Then, we assess the molecular-level regulators of DOM composition across the same set of lakes, identifying mean annual precipitation (MAP), water residence time (WRT) and mean annual temperature (MAT) as major controls. We find that terrestrially derived polyphenols are most abundant in areas with high precipitation and are selectively lost as WRT increases. Furthermore, the abundance of nitrogen (N)-containing compounds increases with MAT. Finally, we evaluate the diversity of DOM molecules in lakes across Sweden and determine the drivers of chemodiversity. We find that the composition and diversity of DOM in Swedish boreal lakes can be explained by climate, hydrology and land use. Distribution of organic molecules in Swedish boreal lakes Sweden presents a unique opportunity to study the effects of environmental gradients on DOM composition in boreal lakes. Over 200,000 lakes pervade the landscape [20] across strong environmental gradients. 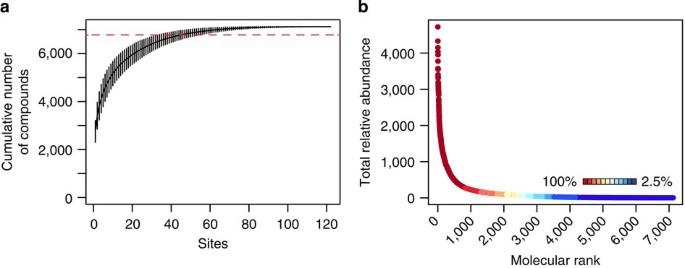Figure 1: Molecular distributions of FT-ICR-MS detected compounds across Swedish lakes. (a) Number of unique molecules with each added lake. Confidence intervals are calculated over 1,000 permutations. The red dotted line indicates 95% of compounds. (b) Rank abundance of the compounds across all lakes shows that the compounds with the highest total relative intensity are most ubiquitous. Molecular compounds are colour coded by the percentage of samples in which they occurred. We studied 120 representative lakes along several environmental gradients across Sweden, for example, MAT (range: −5.2 to 7.5 °C), MAP (range: 450–1,150 mm), in-lake WRT (range: 1–2,000 days) and dissolved organic carbon (DOC) concentration (range: 2.4–51.0 mg l −1 ; see Supplementary Table 1 and Supplementary Fig. 1 for more details). To evaluate the molecular distribution in our dataset, we calculated species accumulation and rank abundance curves using the sum-normalized peak intensities, which from here on we refer to as compounds. Despite the diversity of lakes and the large number of compounds detected in our dataset (totalling 7,122), molecular accumulation across our samples shows a rapid saturation of unique compounds, such that 95% of the molecular richness was reached in 45 of the 120 lakes ( Fig. 1a ). Thus, with each additional sample, fewer previously undetected compounds are identified. For rank abundance analysis, the sum-normalized intensity of each compound was summed across the dataset and then ranked in descending order. Compounds with normalized intensities in the highest 20% are in at least 90% of the samples ( Fig. 1b ), suggesting there is a core of DOM compounds that, while varying in abundance, are ubiquitous throughout the large spatial scale of our study. Figure 1: Molecular distributions of FT-ICR-MS detected compounds across Swedish lakes. ( a ) Number of unique molecules with each added lake. Confidence intervals are calculated over 1,000 permutations. The red dotted line indicates 95% of compounds. ( b ) Rank abundance of the compounds across all lakes shows that the compounds with the highest total relative intensity are most ubiquitous. Molecular compounds are colour coded by the percentage of samples in which they occurred. Full size image Landscape level patterns of organic matter diversity We used non-metric multidimensional scaling (NMDS) to initially assess the relationships between the sum-normalized intensities ( Fig. 2a ), as well as the presence/absence ( Fig. 2b ) of all compounds above the dataset detection limit and environmental gradients. From the pattern of primary variables influencing the distribution of compounds, hydrology emerged as an important driver through the fraction of the watershed of each lake covered by water (% Water), WRT and MAP. Overall, the directions of the influence of these parameters suggest that wet versus dry conditions (for example, shorter versus longer residence time of lakes) result in divergent chemical composition ( Fig. 2 ). Similarly, MAT appears as an important driver, consistent with an opposite correlation to latitude and elevation. These drivers were also identified as highly influential variables when only climate and landscape variables were fit to the NMDS analysis ( Supplementary Fig. 2 ). Several environmental variables were strongly correlated due to their geographical covariance across Sweden, as previously discussed [21] . For instance, % Agriculture is strongly influenced by latitude in this dataset as warmer temperatures and arable soils are most prevalent in southern Sweden. 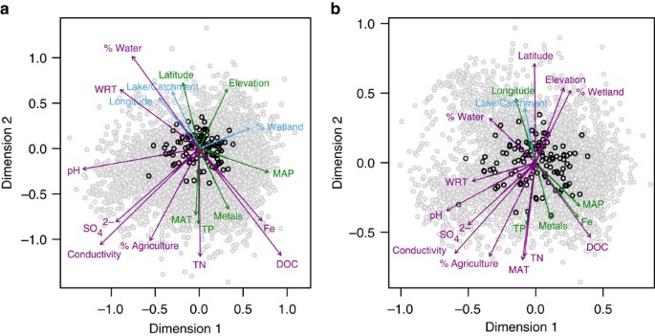Figure 2: Multivariate analysis of molecular data and drivers using non-metric multidimensional scaling. Ordinations are based on either Bray–Curtis (a, stress=0.0966), which utilizes relative compound abundances, or Jaccard distances (b, stress=0.1143), which utilizes presence/absence information. Landscape, climate and in-lake chemistry variables were fit to the ordination. Grey-shaded circles are DOM compounds, whereas black circles indicate the site. Variables with a significance level of <0.05 (light blue), <0.01 (green) and <0.001 (purple) are shown. DOC, dissolved organic carbon; MAP, mean annual precipitation; MAT, mean annual temperature; TN, total nitrogen; TP, total phosphorus; WRT, water residence time. Figure 2: Multivariate analysis of molecular data and drivers using non-metric multidimensional scaling. Ordinations are based on either Bray–Curtis ( a , stress=0.0966), which utilizes relative compound abundances, or Jaccard distances ( b , stress=0.1143), which utilizes presence/absence information. Landscape, climate and in-lake chemistry variables were fit to the ordination. Grey-shaded circles are DOM compounds, whereas black circles indicate the site. Variables with a significance level of <0.05 (light blue), <0.01 (green) and <0.001 (purple) are shown. DOC, dissolved organic carbon; MAP, mean annual precipitation; MAT, mean annual temperature; TN, total nitrogen; TP, total phosphorus; WRT, water residence time. Full size image Linking individual compounds to landscape level drivers We were able to identify the molecular formulae for a total of 4,032 FT-ICR-MS compounds. All detected molecular formulae were categorized into molecular groups, such as polyphenols, polycyclic aromatics or saturated aliphatics (see Methods). Out of these molecules, a subset of 2,500 molecular formulae showed significant variability across the lakes, that is, the variance was at least twice the detection limit, with 981 molecular formulae occurring in 90% of the lakes. Sum-normalized compound intensities were correlated (Spearman rank) to highly influential environmental variables, including MAP, WRT and MAT (see Methods). Across MAP, WRT and MAT, we found clear trends in the molecular composition of DOM ( Fig. 3a–c ). We also restricted our statistical analysis to the more robust subset of 981 molecular formulae that occurred in >90% of the lakes, and the same trends were apparent ( Supplementary Fig. 3 ). In general, we found that the relative abundance of polyphenols increased towards lakes with greater MAP ( Fig. 1a ). Compounds with higher H/C were associated with low MAP, with an inverse pattern observed for WRT ( Fig. 3b ). High MAT was associated with N-containing and oxygenated compounds, whereas low MAT was associated with polyphenols and aliphatic, oxygen-depleted compounds ( Fig. 3c ). Both temperature and hydrology can influence in-lake DOM dynamics [22] , [23] . While warmer temperatures may enhance DOM release from soils [22] , DOM mineralization rates within lakes may also increase [24] . A concurrent decrease in precipitation would reduce transport of terrestrial DOM into aquatic systems and increase WRT in lakes, allowing for greater levels of in-lake processing and reduced DOM concentrations [23] . Advances in FT-ICR-MS data processing now allow us to determine the effects of MAP, WRT and MAT on molecular-level DOM dynamics. 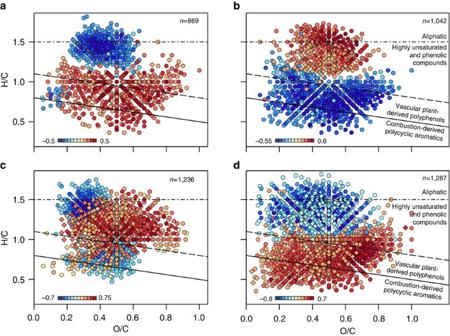Figure 3: Molecular-level DOM patterns across 120 Swedish boreal lakes. Significant Spearman rank correlation coefficients (P-value <0.02674) of individual molecules with (a) mean annual precipitation, (b) water residence time, (c) mean annual temperature and (d) the chemodiversity index. The colour scale indicates Spearman correlations between the intensity of individual molecules and mean annual precipitation, water residence time, mean annual temperature and chemodiversity index (red, positive; blue, negative). Circles indicate compounds without N and diamonds indicate N-containing compounds. Compound groups include combustion-derived polycyclic aromatics (aromaticity index37(AI)>0.66), vascular plant-derived polyphenols (0.66≥AI>0.50), highly unsaturated and phenolic compounds (AI≤0.50 and H/C<1.5), and aliphatic compounds (2.0≥H/C≥1.5). Compound category labels for delineation in panels (b) and (d) also apply to delineated regions in (a) and (c). Lines separating compound categories on van Krevelen diagrams are for visualization only and exact categorization may slightly differ. The number of positive and negative significant correlations can be found inSupplementary Table 2. Figure 3: Molecular-level DOM patterns across 120 Swedish boreal lakes. Significant Spearman rank correlation coefficients ( P -value <0.02674) of individual molecules with ( a ) mean annual precipitation, ( b ) water residence time, ( c ) mean annual temperature and ( d ) the chemodiversity index. The colour scale indicates Spearman correlations between the intensity of individual molecules and mean annual precipitation, water residence time, mean annual temperature and chemodiversity index (red, positive; blue, negative). Circles indicate compounds without N and diamonds indicate N-containing compounds. Compound groups include combustion-derived polycyclic aromatics (aromaticity index [37] (AI)>0.66), vascular plant-derived polyphenols (0.66≥AI>0.50), highly unsaturated and phenolic compounds (AI≤0.50 and H/C<1.5), and aliphatic compounds (2.0≥H/C≥1.5). Compound category labels for delineation in panels ( b ) and ( d ) also apply to delineated regions in ( a ) and ( c ). Lines separating compound categories on van Krevelen diagrams are for visualization only and exact categorization may slightly differ. The number of positive and negative significant correlations can be found in Supplementary Table 2 . Full size image Molecular associations with precipitation and residence time Compounds positively correlated to MAP included combustion-derived compounds and polycyclic aromatics, vascular plant-derived polyphenols and highly unsaturated and phenolic compounds ( Fig. 3a ). The tight association of combustion-derived compounds with plant-derived polyphenols suggests a similar mobilization mechanism from soils, with precipitation-enhanced transport from the catchment [25] . Longer WRT allows for a greater proportion of DOM to be derived from autochthonous sources [21] , [26] and increases photo-exposure. Accordingly, as aromatic compounds are particularly sensitive to photodegradation [11] , we found a decreased abundance of polyphenols with increasing WRT ( Fig. 3b ). This finding is further substantiated by an independent photodegradation experiment on DOM in a tropical river system [13] . Direct comparison of compounds in our study with those from this independent photodegradation experiment [13] revealed that a striking 78% of compounds associated with lower levels of precipitation and 55% of compounds associated with longer WRT in our study were identified as photoresistant [13] ( Fig. 4b,d ). In addition, 64% of compounds associated with high precipitation and 77% of compounds associated with shorter WRT in our study were independently identified as photolabile [13] ( Fig. 4a,c ). The molecular patterns of DOM showed a remarkable coherence between expected history of light exposure in boreal lakes and the photolability of DOM independently described for samples from the Congo River [13] . This not only supports the findings of this study, but also implies the presence of a ubiquitous DOM core that exhibits surprisingly general molecular-level patterns in inland waters, across biomes and continents. 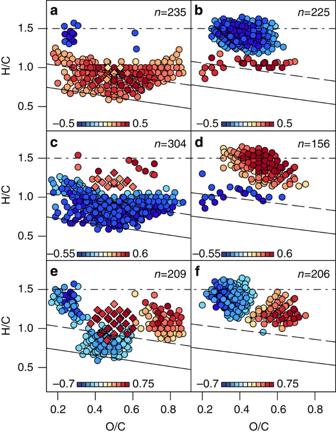Figure 4: Comparison of molecular-level patterns driven by landscape scale parameters and photoreactivity. Compounds found in ≥90% of our lakes that significantly correlated with mean annual precipitation, water residence time or mean annual temperature and that were experimentally identified13as photolabile or photoresistant in the Congo River. The colour scale indicates the strength and direction of the significant (P-value <0.02674) molecule-specific Spearman correlations with mean annual precipitation (a,b), water residence time (c,d) and mean annual temperature (e,f), but grouped and independently identified as photolabile (a,cande) or photoresistant (b,dandf)13. Circles and diamonds indicate N-free and N-containing compounds, respectively. Most compounds that correlated positively with mean annual precipitation were identified as photolabile, and most compounds negatively correlated with mean annual precipitation were photoresistant. The inverse was observed for water residence time. Compound groups include combustion-derived polycyclic aromatics (aromaticity index37(AI)>0.66), vascular plant-derived polyphenols (0.66≥AI>0.50), highly unsaturated and phenolic compounds (AI≤0.50 and H/C<1.5), and aliphatic compounds (2.0≥H/C≥1.5). The number of positive and negative significant correlations can be found inSupplementary Table 2. Figure 4: Comparison of molecular-level patterns driven by landscape scale parameters and photoreactivity. Compounds found in ≥90% of our lakes that significantly correlated with mean annual precipitation, water residence time or mean annual temperature and that were experimentally identified [13] as photolabile or photoresistant in the Congo River. The colour scale indicates the strength and direction of the significant ( P -value <0.02674) molecule-specific Spearman correlations with mean annual precipitation ( a , b ), water residence time ( c , d ) and mean annual temperature ( e , f ), but grouped and independently identified as photolabile ( a , c and e ) or photoresistant ( b , d and f ) [13] . Circles and diamonds indicate N-free and N-containing compounds, respectively. Most compounds that correlated positively with mean annual precipitation were identified as photolabile, and most compounds negatively correlated with mean annual precipitation were photoresistant. The inverse was observed for water residence time. Compound groups include combustion-derived polycyclic aromatics (aromaticity index [37] (AI)>0.66), vascular plant-derived polyphenols (0.66≥AI>0.50), highly unsaturated and phenolic compounds (AI≤0.50 and H/C<1.5), and aliphatic compounds (2.0≥H/C≥1.5). The number of positive and negative significant correlations can be found in Supplementary Table 2 . Full size image Despite the consistency of molecular-level patterns within compound groups, highly unsaturated and phenolic compounds, with formulae typical of lignin, tannin and carboxylic-rich alicyclic molecules [15] , show an overt shift in molecular associations with MAP and WRT just above H/C=1 ( Fig. 3a,b ). More unsaturated compounds were positively related to MAP whereas more aliphatic compounds were negatively associated to MAP, with a clear inverse pattern observed for WRT. This defined shift in molecular patterns associated with MAP and WRT suggests a transition at H/C≈1 between aromatic, photoreactive compounds and those resistant to photolysis. Molecular associations with MAT MAT presents a less straightforward association with DOM across Sweden ( Fig. 3c ). N-containing compounds were positively correlated to MAT, suggesting greater abundance where temperatures are higher and agriculture is more prevalent. A majority (65%) of N-containing compounds positively correlated to MAT were also positively correlated to residence time. Longer WRT increases the attenuation of DOM [27] , particularly DOM of terrestrial origin, thus increasing the relative importance of in-lake produced DOM [21] , [26] . While the proportion of autochthonous carbon will increase, the actual in-situ production is 1-2 orders of magnitude less than that from terrestrial import in Swedish boreal lakes [10] . An additional 31% of N-containing compounds positively associated with MAT, but not significantly correlated to WRT, were positively associated with MAP. While this suggests a catchment origin, a positive correlation with MAP may reflect inorganic nutrient additions and a consequent autochthonous production of organic N. A group of aliphatic, but oxygen-depleted compounds were negatively associated with MAT, prevalent in northern Sweden where the MAT is markedly lower than southern Sweden (mean±s.e. : −1.8±0.3 and 5.4±0.1 °C, respectively). A majority (70%) of these aliphatic, but oxygen-depleted compounds negatively associated with MAT were negatively correlated to MAP. With MAT well below freezing in northern Sweden, transport from the landscape is highly constrained [25] , which could result in a greater relative abundance of aliphatic compounds produced within the lakes. For more southern lakes with MAT above freezing, these aliphatic compounds could be dwarfed by terrestrial imports [24] or rapidly degraded, reflecting the constraints of DOM processing at below zero MATs [28] . Regulators and molecular associations of chemodiversity While DOM composition reflects variation in MAP, WRT and MAT, chemodiversity was most strongly correlated to concentrations of organic carbon (Spearman correlation: 0.36, P <0.0001) and total N (Spearman correlation: 0.30, P =0.0007). The chemodiversity of DOM in each lake was calculated using the Chao 1 diversity index [29] , considering each compound as a chemical species. Lakes with lower chemodiversity contained fewer aromatic but more aliphatic compounds ( Fig. 3d ), whereas compounds with a H/C≤1, primarily vascular plant-derived polyphenols and combustion-derived polycyclic aromatics, were associated with higher chemodiversity. Our results suggest that lakes with high DOC concentrations contain the most diverse mixture of recently imported terrestrially derived DOM. Chemodiversity is then reduced as in-lake processes, for example, photodegradation and sedimentation via flocculation, preferentially remove the colored fraction of terrestrially derived DOM [26] . A high association with total nutrients suggests that nutrient import from the catchment promotes chemodiversity, enhancing in-lake production and transformation of DOM. Total phosphorus was not significantly correlated to chemodiversity, possibly a consequence of frequent N-limitation observed in hyper-oligotrophic northern lakes [30] . Nonetheless, nutrients are washed in from the catchment, along with terrestrial DOM, highlighting the importance of catchment properties such as land use in enhancing chemodiversity. Climate scenarios for Sweden and the boreal zone generally predict a warmer and wetter climate [31] , with changes in MAP affecting WRT and, along with changes in MAT and land use, ultimately affecting the current distribution of chemodiversity. Thus, in areas experiencing increases in MAP, our study suggests the abundance of polyphenols will increase, diminishing the influence of in-lake processing on DOM quality. An increase in vascular plant-derived polyphenols in lakes would reduce light penetration, oxygen penetration and stratification depths [32] , increase heterotrophy [5] , [10] and decrease overall productivity [6] , with changes in the quality of DOM in source waters having clear implications for drinking water treatment [33] . Furthermore, increased delivery of polyphenols to coastal areas could increase light-mediated bacterial production [19] , straining areas that are already O 2 limited. Alternatively, in areas with declining MAP, aliphatic compounds would increase in relative abundance, a consequence of decreasing discharge and increasing WRT. This would simultaneously enhance both the degradation of imported unsaturated, polyphenolic and condensed polyaromatic DOM and the in-lake production of aliphatic compounds [13] , [21] , [26] . Qualitative differences due to changes in MAT are likely to be greatest in areas shifting from MATs below to above freezing. With increased MAT projected across Sweden [31] , or with changes in land use, the prevalence of N-containing and unsaturated, oxygenated compounds is likely to increase. Lakes have a disproportionately large influence on the processing of organic carbon as it is transported to the ocean [7] , [8] , [9] , [10] . This study demonstrates that qualitative changes in DOM are largely driven by broad-scale climatic variables, hydrology, organic matter and nutrients. As broad-scale climatic variables can be used to elucidate molecular-level patterns, independently of local variables (for example, soil type and vegetation), predictions of how DOM quality will change in response to climate change are increasingly feasible. Sample collection and FT-ICR-MS sample preparation Lake water samples were collected by helicopter from 120 lakes distributed across Sweden ( Supplementary Fig. 1 ) at 1-m-depth within a 2-month period (September 26–November 25, 2010) as part of the Swedish Environmental Protection Agency’s lake monitoring programme. Water chemistry (total organic carbon, pH, alkalinity, conductivity, nutrients, and metal and non-metal ions) was analyzed according to standard methods. Sampling and chemical analysis was conducted at the Department of Aquatic Sciences and Assessment, Swedish University of Agricultural Sciences (SLU) [34] . MAT and MAP were derived from data collected by the Swedish Meteorological and Hydrological Institute. Lake specific MAT was calculated by correcting for elevation using the relationship −0.6 °C per 100 m (ref. 35 ). Samples were filtered with 0.45 μm mixed cellulose ester membranes (GN-6 Metricel, Pall Life Sciences), and kept at 4 °C until solid-phase extraction in January 2011. DOM was extracted using 100 mg Bond Elut PPL cartridges (Agilent Technologies) [36] to remove salt and limit artifacts created in FT-ICR-MS by differences in DOM concentrations across our wide range of samples. The volume passed over the sample was adjusted based on DOC concentration, so that the eluate would have a target concentration of 20 mg C l −1 . Acidified sample (pH 2) was passed over the cartridge, rinsed with two cartridge volumes of 0.01 N HCl, and dried with ultrapure He gas. After the cartridges were completely dry, DOM was collected from the solid phase using LC-MS Chromasolv grade methanol (Sigma-Aldrich). Extraction efficiency (69±8% on average, n =8) was calculated for a subset of samples by drying an aliquot of methanol eluate, redissolving it in ultrapure water and measuring the DOC concentration on a Shimadzu TOC analyzer (V series). Eluates were stored at −20 °C in acid washed and combusted amber glass vials until being prepared for analysis on a FT-ICR-MS (Bruker Daltonics, Bremen, Germany) in Oldenburg, Germany. Methanol eluates were diluted 1:1 (v/v) with ultrapure water. The samples were refiltered with 0.2 μm PTFE syringe filters prerinsed with a 1:1 mixture of methanol to ultrapure water immediately preceding analysis on the FT-ICR-MS. FT-ICR-MS analysis Negative ions of DOM eluates were produced via electrospray ionization and the complex molecular character of freshwater DOM was subsequently analyzed using a 15 T ultrahigh-resolution FT-ICR-MS. Samples were injected at a rate of 120 μl h −1 . The capillary and spray shield voltages were 4,000 and −500 V, respectively, and the drying gas had a flow rate of 3.7 l min −1 at 200 °C. Mass spectra were collected over 500 scans, with an ion accumulation time of 0.6 s, a time of flight of 0.55 s and a range of 150–2,000 m/z . No peaks occurred above 1,000 m/z . Molecular formulae were assigned to peaks with a signal to noise ratio greater than four, according to stringent criteria with elemental combinations of C 1–100 H 1–250 O 1–100 N 0–4 P 0–1 S 0–1 (ref. 16 ). Molecules with extreme heteroatom assignments (with N =4 and S=1) were excluded from the data. No systematic trends in P-containing compounds, S-containing compounds or N-containing compounds with N >2 were observed across the lakes, thus these compounds were not included in the discussion. Peaks were considered with a signal to noise ratio greater than four. FT-ICR-MS signal intensities were normalized to the sum of all signals (sum-normalized intensity) after removing peaks detected in procedural blanks. Peaks in fewer than four samples were not considered. To compare such a diverse sample set, we then set a threshold, or the dataset detection limit, where all peaks with a sum-normalized intensity lower than the smallest peak (S/N>4) in the sample with the worst resolution are not considered. Sum-normalized intensities between the dataset detection limit and two times the detection limit, or the threshold of determination, were given a value of 1.5 times the detection limit. This peak processing method resulted in a dataset of 7,122 peaks, with 4,032 peaks (57%) having formula assignments. Number of peaks in each sample ranged from 2,235–3,308, and formulas could be assigned to 69.3±3.4% (average±s.d.) of the peaks in each sample. The majority of unassigned peaks (53%) were not ubiquitous, occurring in 10% of samples or less. Molecules were assigned to compound groups based on the stoichiometry of their molecular formula. The groups relevant to our study are delineated by the aromaticity index (AI) [37] , [38] and H/C cutoffs [38] : combustion-derived polycyclic aromatics (AI>0.66), vascular plant-derived polyphenols (0.66≥AI>0.50), highly unsaturated and phenolic compounds (AI≤0.50 and H/C<1.5), and aliphatic compounds (2.0≥H/C≥1.5). Molecular distributions and multivariate analysis Species accumulation, rank abundance and NMDS were calculated on the sum-normalized intensity of all compounds above the dataset detection limit, including compounds where the formulae could not be assigned, that occurred in at least three samples (totalling 7,122 peaks). The species accumulation curve was calculated adding the samples in a random order with 1,000 permutations, showing 95% confidence intervals. This calculation gives a confidence interval for the number of unique compounds detected with each additional sample. Rank abundance shows the molecules with the sum of sum-normalized peak intensities across samples in descending order. The color represents the percentage of samples in which each compound occurred. NMDS was calculated using relative peak abundances (Bray-Curtis; Fig. 2a and Supplementary Fig. 2a ; stress=0.0966) and presence/absence (Jaccard; Fig. 2b and Supplementary Fig. 2b ; stress=0.1143). Landscape, climate and in-lake chemistry variables were fit to each ordination, with P -values calculated over 999 permutations ( Fig. 2 ). Landscape and climate variables were also fit to each NMDS independently from chemistry variables, with P -values calculated over 999 permutations ( Supplementary Fig. 2 ). Species accumulation and NMDS were calculated using the R software package vegan [39] , and the rank abundance curve was calculated using the R software package BiodiversityR [40] . Molecular correlations with environmental parameters Patterns of molecular associations with climate, hydrology, land use and water chemistry were tested using Spearman’s rank correlation coefficient (Spearman correlation). The Spearman correlation is a non-parametric measure of how strongly two variables are related to one another, with reduced sensitivity to outliers and no assumptions on the distribution of the measurements. This allows for the inclusion of parameters that are not normally distributed, however reducing the power of the analysis, as the Spearman correlation is more conservative than Pearson’s correlation coefficient. The Spearman correlation was calculated between environmental parameters and the sum-normalized intensity of peaks where the formulae could be unambiguously assigned, that were present in at least 90% of the samples and where intensity of the peak was greater than the limit of determination in at least half of the samples ( n =981, Supplementary Figs 3, 4 ). These criteria were set to see how molecules change across environmental parameters. This conservative approach was taken to increase confidence in our findings and to avoid highlighting spurious or weak correlations that are only significant due to the large sample size. This conservative approach reveals distinct and major molecular patterns across environmental variables ( Supplementary Fig. 3 ), and adds weight to the same patterns observed across less stringent correlation criteria. Less stringent criteria (formulae were included that were found in more than three samples and where the minimum variance was greater than twice the detection limit, n =2,500) revealed the same molecular trends across MAP, WRT, MAT and chemodiversity with a greater number of significant correlations ( Fig. 3 ). The high agreement between the systematic patterns found in both our more conservative and less stringent approaches suggests that the molecular-level patterns observed apply to many more compounds than just a DOM core abundant in most lakes. To correct for the large number of tests performed, we applied a false discovery rate correction [41] , which adjusted the maximum original P -value considered significant to P <0.02674. The aim of using a false discovery rate correction is to control the fraction of Type I errors, without unnecessarily increasing the risk of Type II errors. The environmental parameters covered climate (MAT and MAP), land cover (% Agriculture, % Forest, % Wetland, % Water and % Other), hydrology (slope, runoff, WRT, lake/catchment area, surface area and volume), geography (elevation, latitude and longitude), and water chemistry (DOC, pH, conductivity, total nitrogen, total phosphorus, SO 4 2− , iron (Fe) and the sum of transition metals (As, Cd, Co, Cr, Cu, K, Mn, Ni, Pb, Si, V, Zn)). Spearman correlations were then plotted in a van Krevelen space [42] for each environmental parameter, major patterns of molecular variation were visually identified, and variables were grouped based on similar patterns of correlations. The large-scale variables MAP and MAT and WRT described major molecular patterns across our dataset ( Figs 2 , 3 and Supplementary Fig. 3 ), as well as drive many of the patterns observed with other measurements. The selection of these external drivers was validated by NMDS on the mass spectra peaks with environmental variables fit to the NMDS. Reproducibility and duplicate analysis While peak intensities in FT-ICR-MS analyses cannot directly be related to concentrations across a wide assortment of samples, all samples were solid phase extracted in a random order, following the same protocol. Extracting the same amount of DOM from each sample mitigated artifacts resulting from differences in DOC concentrations in the eluates. Additionally, all samples were run on the same FT-ICR-MS, which has previously shown high reproducibility of replicates [43] , in a random order and with the same settings. Therefore, all samples are biased in the same way and not along any particular gradient (for example, DOC concentration). Furthermore, we ran an in-house reference sample from the deep North Pacific at the beginning and end of each day. We tested the correlation of the intensities of all peaks above the dataset detection limit between each pair of replicates using Pearson’s correlation. The average Pearson correlation and standard deviation across replicates were then calculated. The reproducibility of the reference sample was very high (average r ±s.d., 0.98±0.01). We analyzed sample replicates in the same way: the average correlation (±s.d.) between replicates was 0.97 (±0.03, n =31 (26% of the dataset)), again confirming the reproducibility of the sum-normalized peak intensity across our dataset. Using normalized peak intensities as opposed to presence/absence-based methods broadens the range of statistical tools available to study and interpret DOM patterns. In accordance with a previous study [44] , we find that utilizing normalized peak intensities reveals more detailed patterns and drivers of DOM quality than were apparent from only using presence/absence information, in both multivariate analyses ( Fig. 2 and Supplementary Fig. 2 ) and univariate analyses ( Fig. 3 and Supplementary Fig. 3 ). Chemodiversity Index The chemodiversity index was calculated as the richness estimator Chao 1 (ref. 29 ), using the R software package vegan [39] , with the individual compounds as species and the relative intensity of the peaks used as species abundance. We rounded the sum-normalized peak intensities in each sample so the peak intensities would mimic species counts, thus the minimum value in each sample was 1. These peaks can then be considered singletons (and peaks with a value of 2, doubletons) in each sample. Chao 1 uses singletons and doubletons in a sample to estimate the minimum unobserved richness of a sample. If a sample has many rare compounds, more singletons would be measured, suggesting there are more rare compounds that have not yet been measured. The absence of singletons implies no rare species are left unmeasured. This is a suitable measure for chemodiversity as FT-ICR-MS data contains many peaks that may be excluded if they fall under the signal to noise ratio or detection limit applied. After the chemodiversity index was calculated for each sample, associations between environmental parameters and the chemodiversity index were tested using Spearman’s correlation to look for possible associations between DOM diversity and climate, landscape variables and water chemistry. Then Spearman’s correlation was utilized to identify compounds that are associated with the chemodiversity index. These relationships were again plotted in a van Krevelen space to further interpret the relationships between molecules and molecular diversity. How to cite this article: Kellerman, A. M. et al. Chemodiversity of dissolved organic matter in lakes driven by climate and hydrology. Nat. Commun. 5:3804 doi: 10.1038/ncomms4804 (2014).